Lightweight nanoporous metal hydroxide-rich zeotypes Nanoporous materials have important industrial applications as molecular sieves, catalysts and in gas separation and storage. They are normally produced as moderately dense silicates (SiO 2 ) and aluminosilicates making their specific capacities for the uptake and storage of gases, such as hydrogen, relatively low. Here we report the synthesis and characterization of lightweight, nanoporous structures formed from the metal hydroxide Be(OH) 2 in combination with relatively low levels of framework phosphate or arsenate. Three new zeotype structures are described, constructed mainly of Be(OH) 4 tetrahedra bridged through hydroxide into three-membered rings; these units link together to produce several previously unknown zeotype cage types and some of the most structurally complex, nanoporous materials ever discovered. These materials have very low densities between 1.12 and 1.37 g cm −3 and theoretical porosities of 63–68% of their total volume thereby yielding very high total specific pore volumes of up to 0.60 cm 3 g −1 . The discovery of new inorganic framework materials that exhibit microporosity is an important synthesis target as has been recently highlighted [1] , [2] , [3] , [4] , [5] , [6] , [7] . The widespread industrial use of zeolites and zeotypes in areas as diverse as catalysis, gas separation and storage, ion exchange and as desiccants requires the design and control of structural and chemical properties such as pore size and interconnectivity, thermal stability, surface site acidity, chirality and, for gas storage, weight. The incorporation of species beyond silicon and aluminium onto the tetrahedral sites in zeotype materials often yields improved functionality and new pore types and topologies with different characteristics for catalysis. For instance aluminophosphates (AlPOs, general formula AlPO 4 and isomorphic with SiO 2 ) are used widely in base catalysis conditions [8] . Related areas of research involve the use of organic linking species and centre on the development of metal-organic frameworks (MOFs); examples of the compounds synthesized under this heading include MIL-101 (refs 9 , 10 ), covalent organic frameworks [11] , zeolitic imidazolate frameworks [12] and lightweight beryllium-based MOFs [13] . For gas storage applications, where high specific gas uptakes are needed, zeolites and AlPOs offer the high nanoporosities and internal surface areas required; however, the presence of the second row elements, silicon, aluminium and phosphorus, yields moderate compound densities of, typically, 2–3 g cm −3 . As a result the best theoretical specific hydrogen gas uptakes in zeotypes are typically reported as only 2–4wt% (ref. 14 ) and measured values at 77 K in Na-Y at 2.55wt% (ref. 15 ). Some MOFs and related phases have very large internal volumes but their low internal surface areas means that gas uptake is mainly by weak physisorption and, therefore, only occurs at near theoretical values just above the gas liquefaction temperature or at high pressures at 77 K (ref. 16 ). Ultra-lightweight materials include carbon nanotube aerogels [17] , metallic microlattices [18] and silica xerogels [19] , all with densities <10 mg cm −3 ; however, these structured materials do not grow in crystalline forms and their internal surface areas for strong physisorption are relatively low. For catalytic processes, the dimensions and dimensionality of the zeotype pore system are key parameters so that important targets in zeotype synthesis are new channel and cage topologies, and the control of their connectivity. The number and nature of Brönsted (T-OH-T, T = Si, P, Al, etc) or Lewis acid sites also have important effects on the performance of a zeotype catalyst [20] with high Brönsted acidities keenly sort after. The flexibility in linking TO 4 tetrahedra gives rise to over 200 zeotypes many of which, in purely silaceous forms constructed only of SiO 4 tetrahedra, are considered as SiO 2 polymorphs [21] . Other TX 4 units which when fully linked three dimensionally produce TX 2 stoichiometries include [Be(OH) 4 ], as in β-Be(OH) 2 with the Zn(OH) 2 structure type [22] . This presents the intriguing possibility of producing porous zeotype analogues of the stoichiometry 'Be(OH) 2 ', which, because of the low atomic mass of beryllium, would be of significantly lower density than silicon-based structures; materials of this type should also have extremely high levels of strongly acidic Brönsted acid sites, T-OH-T. Previously reported zeotypes containing some BeO 4 tetrahedra include beryllosilicates, beryllophosphates and beylloarsenates [23] , [24] , [25] , [26] . The majority of these do not demonstrate Be:T' ratios (where T' is Si, P or As) above unity partly because, with oxygen as the bridging anion, the framework would develop a very high negative charge and the bridging oxygen is under-bonded when connected solely to two Be 2+ ions. However, examples of frameworks with Be:T' >1 exist in the naturally occurring mineral Weinebenite CaBe 3 (PO 4 ) 2 (OH) 2 •4H 2 O [27] and the recently reported [NH 4 ] 2 [As 2 Be 3 O 8 (OH) 2 ], both with Be:T'=1.5 (ref. 26 ). These compounds achieve the higher ratio by partially employing OH − anions as the bridging group between two Be-centred tetrahedra as in β-Be(OH) 2 ; the existence of this structural feature provides a basis by which high levels of beryllium might be incorporated into zeotypes. Here we report three new beryllium-rich zeotype framework topologies with stoichiometries approaching Be(OH) 2 yielding low framework densities (FDs, tetrahedra per 1000 Å 3 ) and very low specific material densities near 1.1 g cm −3 (beryllophosphate) and 1.3 g cm −3 (berylloarsenates). These complex topologies, formed mainly of spiro-5 rings and new cage types, also include some of the most structurally complex zeotypes discovered. A comprehensive investigation of beryllium–arsenate and beryllium–phosphate framework chemistry was undertaken using a variety of amine templates to induce nanoporous structure formation. Overall 21 new berylloarsenates were obtained and structurally characterized and 10 new beryllophosphates. A few of these berylloarsenates have been reported previously [26] ; this communication focuses on three new, fully-connected (zeotype), high-porosity, beryllium-rich beryllophosphate and berylloarsenate frameworks. Beryllium framework ten Beryllium framework ten (BET) was found for both beryllophosphate [C 2 H 5 NH 2, H 2 O] x [ Be~ 72 P~ 20 (O)~ 60 (OH)~ 124 ]=[Be~ 0.78 P~ 0.22 (O,OH) 2 ] (BET-P) and berylloarsenate [C 2 H 5 NH 2, H 2 O] x [Be 66.7 As 25.3 (O) 80.5 (OH) 103.5 ]=[Be 0.72 P 0.28 (O,OH) 2 ] (BET-As) compositions, crystallizing with cell volumes of 6524 and 6894 Å 3 respectively. Beryllium and phosphorus/arsenic are distributed over the T-atom sites with individual site Be:P/As ratios ranging from near 1.0:0.0 to 0.5:0.5 producing overall ratios of 3(±0.3):1 (BET-P) and 2.5(±0.15):1 (BET-As). For charge balance the bridging anion is a mixture of O 2− and, predominately, OH − . The most common, simple secondary building unit is the spiro-5 ring (lov), formed from two 3-rings with a common central tetrahedron, though one single four-ring is present in the asymmetric unit cell. The structure is formed of sinusoidal chains of spiro-5 rings along a lattice direction that are further connected to produce a complex network of two unusual cage types: 10 2 -8 5 -3 10 pentagonal drum-shaped cages (formed by two parallel ten-membered rings (10Rs) connected by their edges through five spiro-5 rings), hereafter termed ben, and an asymmetric cage (termed bet) formed from 8 4 -6 2 -4 1 -3 6 rings, Fig. 1a,b . Neighbouring ben and bet cages form columns running through the structure along the c crystallographic axis generating linear channels of 10Rs along the a axis and 8Rs along the c axis. Each network in the ac plane is connected to the next layer by spiro-5 rings, which emanate from the bet cages in the adjacent layer and join with a ben type cage producing the sequence bet–lov–ben–bet along the b axis. The connectivity between the network layers in the ac plane results in interconnected 10R channels along 101 and 10-1 directions ( Fig. 1c,d ; Supplementary Fig. S1a,b ). 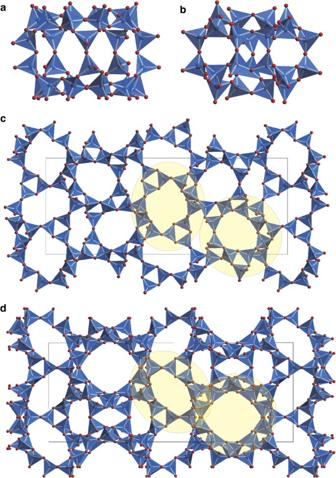Figure 1: The BET structure type. The (a) ben and (b) bet cages. (c) The structure viewed down the a axis and (d) depicts the view down the c axis. The unit cell is outlined in black. The (Be,As,P)(O,OH)4tetrahedra are shaded blue and oxygen atoms are shown as red spheres. One position of each of the ben and bet cages is outlined with pale yellow shading in each view, as an ellipse and a circle, respectively. Figure 1: The BET structure type. The ( a ) ben and ( b ) bet cages. ( c ) The structure viewed down the a axis and ( d ) depicts the view down the c axis. The unit cell is outlined in black. The (Be,As,P)(O,OH) 4 tetrahedra are shaded blue and oxygen atoms are shown as red spheres. One position of each of the ben and bet cages is outlined with pale yellow shading in each view, as an ellipse and a circle, respectively. Full size image Beryllium framework eleven Beryllium framework eleven (BEE), [R + ] 1.5 [As 6.17 Be 13.83 O~ 20 OH ~20 ]. n H 2 O, crystallizes from solution under hydrothermal conditions in combination with beryllium framework one-two (BOT; vide infra), Fig. 2 , and its complex unit cell ( V =9031 Å 3 ) contains 30 unique T-atom sites; the majority are purely beryllium centred and residue mixed Be/As. BEE is formed solely of spiro-5 rings (lov), which connect to form the ben cages seen in BET. The cages are aligned to produce almost linear and slightly zig–zag 10R and 8R channels along both the b and a directions. These channels are mainly interconnected through a further distorted 8R aperature along the 101 direction to form a fully interconnected three-dimensional pore and channel system; however, one linear 10-ring channel along the b axis is independent of this main channel system ( Supplementary Fig. S1c,d ). 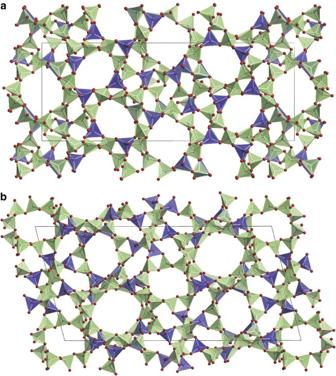Figure 2: The BEE structure type. (a) The structure viewed down the a axis and (b) depicts the view along the c axis. The unit cell is outlined in black. (Be,As)(O,OH)4tetrahedra are shaded green (those purely or very predominantly beryllium-centred) and purple (30% or greater arsenic-centred). Figure 2: The BEE structure type. ( a ) The structure viewed down the a axis and ( b ) depicts the view along the c axis. The unit cell is outlined in black. (Be,As)(O,OH) 4 tetrahedra are shaded green (those purely or very predominantly beryllium-centred) and purple (30% or greater arsenic-centred). Full size image Beryllium framework one-two The structure of BOT, [C 2 H 5 NH 2 ][Be 42.7 As 17.3 (O)~ 55 (OH)~ 65 ], was solved in the orthorhombic Cmcm space group with a highly disordered Be and As distribution; localized ordering of these T atoms and the associated bridging O,OH anions is likely to occur such that the true symmetry of the structure is lower than orthorhombic. BOT, in common with BEE, is entirely constructed of spiro-5 rings, which form, in the ac plane, complex networks of sinusoidal chains of rectangular 10Rs running along c ( Fig. 3a–c ; Supplementary Fig. S1e ). These 10Rs are connected along the a axis direction by 8Rs, which present an almost square profile when viewed down this crystallographic axis. Each network in the ac plane is connected to the next by spiro-5 rings, which produce interconnecting 10R apertures along both the a and c directions. At the intersection of these 10Rs, a new type of large zeotype cage is formed from 10 4 -8 2 -4 2 -3 10 rings with the four 10Rs connected through eight 3Rs on to a base of two 8Rs and two 4Rs, Fig. 3d . 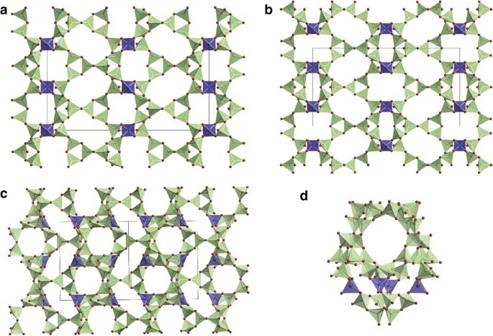Figure 3: The BOT structure type. (a) The structure viewed down the a axis, (b) the view along the c axis and (c) the channel system that exists along the 110 direction. The unit cell is outlined in black. (Be,As)(O,OH)4tetrahedra are shaded green (those purely or very predominantly beryllium-centred) and purple (30% or greater arsenic-centred). (d) The new large zeotype cage found in BOT consisting of the rings 104-82-42-310. Figure 3: The BOT structure type. ( a ) The structure viewed down the a axis, ( b ) the view along the c axis and ( c ) the channel system that exists along the 110 direction. The unit cell is outlined in black. (Be,As)(O,OH) 4 tetrahedra are shaded green (those purely or very predominantly beryllium-centred) and purple (30% or greater arsenic-centred). ( d ) The new large zeotype cage found in BOT consisting of the rings 10 4 -8 2 -4 2 -3 10 . Full size image Comparison of the new framework structures Consideration of the structures of these three new frameworks shows a number of features in common. The main building unit is the spiro-5-ring consisting of apex-linked 3-rings, a feature that is prevalent in zeotypes containing Be(O,OH) 4 units; the high proportion of beryllium on T sites found in BET, BEE and BOT, at around 70%, leads to the observed dominance of this structural building unit. As a result linkages of the type Be-OH-Be with bridging hydroxide are dominant in these zeotypes; linking through oxide would leave this anion strongly under-bonded with just two neighbouring divalent Be centres. Bridging hydroxide is found at low levels in the zeotype mineral Weinebenite CaBe 3 (PO 4 ) 2 (OH) 2 •4H 2 O [27] , where the 3Rs containing two BeX 4 tetrahedra are linked through Be-OH-Be, and several other synthetic zeotypes such as -WEN, -ITV, -UEI, -RON and -LIT [28] . Porosities of the new frameworks Theoretical porosities were calculated using the ZEOMICS package [29] and are presented in Table 2 in comparison with several well-known zeolites. Experimental measurements of thermal stability (thermogravimetric analysis, TGA ; Supplementary Fig. S2 ), molecular adsorption and porosity ( Supplementary Fig. S3 ) were undertaken on BET-As, as this could be produced as a high-purity single phase; BEE and BOT invariably grew as a polyphasic mixture with small levels of an amorphous phase visible under optical magnification. Variable temperature powder X-ray diffraction (PXD) data showed that BET-As starts to lose framework integrity when heated above 250 °C ( Supplementary Figs S4 and S5 ). Weight loss data from TGA and levels of water and template molecules estimated from residual extra-framework electron density extracted from SQUEEZE yield a synthesized composition of [C 2 H 5 NH 2, H 2 O] 120 [Be 66.7 As 25.3 (O) 80.5 (OH) 103.5 ]; a level of hydration similar to that found for zeolite-X (FAU), which has a similar pore volume. Approximately 80% of the extra-framework material can be removed from BET-As before the structure collapses; a similar level to that found in many other zeolites. For BET-As a total pore volume of 0.36 cm 3 g −1 was determined ( Supplementary Fig. S3 ), a value about that half that expected from theory; surface area measurements using material from which water and templating molecules have not been fully removed invariably give reduced values due to the lower available volume and pore blocking. Acidity of the OH units in BET-As was probed by infrared spectroscopy [30] , [31] and pyridine adsorption ( Supplementary Fig. S6 ). The framework OH-stretch is located at 3479 cm −1 , a value similar to that found for Be(OH) 2 and one that indicates that these protons are highly acidic in comparison with those in the Brønsted acid forms of aluminosilicate zeolites, which typically absorb near 3600 cm −1 (ref. 31 ). The aim of this work was to investigate whether hydroxides of the composition M(OH) 2 could replicate the chemistry seen with SiO 2 in highly siliceous zeolites, such as MFI silicalite [32] and siliceous ZSM-12 (MTW topology) [33] . The high levels of beryllium present in the frameworks found in this work, Table 1 , leads to OH − :O 2− ratios greater than unity, such that the stoichiometry of each of these frameworks tends towards a nanoporous polymorph of Be(OH) 2 . In addition a high level of 3Rs in a zeotype structure is known to lead to a low FD, the number of tetrahedral atoms ( T ) per 1000 Å 3 ; this is exemplified by the beryllosilicate zeotypes OSO and OBW with FDs of 13.3 and 12.7, respectively [23] . Table 1 also summarizes the FDs of the BET, BEE and BOT structures, which show the expected low values. Indeed the value for BOT is one of the lowest known for a fully connected oxoanion framework at 12.6 T atoms per 1000 Å 3 , a value even more remarkable given the relatively short, for zeotypes, average T-O distance of ~1.65 Å. These low FDs result from the high proportion of two- and three-dimensionally, interconnected, new cage units, such as ben and bet, with intersecting 10R channels ( Fig. 1a,b and Supplementary Fig. S1 ), a feature of note in zeolite-catalysed methanol to hydrocarbon reactions [34] . Table 1 Summary of framework parameters. Full size table The low FDs coupled with the high Be:P and Be:As ratios result in very low material densities, as summarized in Table 1 , with the BET-P and beryllium-rich, highly porous structure of the berylloarsenate BOT yielding the lowest values of 1.12 and 1.27 g cm −3 , respectively. These results point to what is achievable with frameworks constructed with very light atom centred polyhedra. For example, the BOT framework with purely beryllium-based tetrahedral as a Be(OH) 2 polymorph would have a density of only 0.88 g cm −3 ; while replacing As by P at the levels found in BET-P would decrease its density to near 1 g cm −3 . Although such values are significantly higher than many large pore MOFs and meso-structured, ultra-lightweight materials [16] , [17] , [18] , [19] , a key feature of these beryllium hydroxide-based frameworks is that the high internal surface area is likely to be available for the strong physisorption of gases. Even within the larger cage sizes, such as bet, the maximum wall-to-wall separation is 10.2 Å, and allowing for partial decoration of these walls by OH groups reduces these distances further. The materials demonstrate large theoretical pore volumes of around 65–70%, Table 2 . For a purely siliceous framework, this yields respectable total pore volumes of more than 0.5 cm 3 g −1 and for as-synthesized BET-P a value of 0.60 cm 3 g −1 ; for a pure Be(OH) 2 composition with the BOT structure, a total pore volume of 0.763 cm 3 g −1 and surface area (2 Å characteristic molecular diameter) of 2247 m 2 g −1 can be calculated. This specific pore volume is about twice that of a typical aluminosilicate zeolite and corresponds to an idealized hydrogen uptake of 5.4wt%—far higher than those of the aluminosilicate zeolites [35] . Although the experimentally determined nitrogen uptake for framework BET-As is much lower, probably, because of incomplete dehydration under thermal conditions that do not start a collapse of the framework, respectable experimental uptakes of 0.36 cm 3 g −1 were observed. Other methods of extracting water and template molecules from these materials such as freeze vacuum drying are under investigation. Table 2 Porosity data for the new zeotypes and known zeolites calculated using ZEOMICS(29). Full size table Although the toxicity of beryllium may limit the application of beryllium hydroxide zeotypes to specialized applications where weight is the primary concern, e.g., spaceflight, it is noteworthy that the structure of LiB(OH) 4 consists of linked Li(OH) 4 and B(OH) 4 tetrahedra [36] . Many zeotype aluminium phosphates (AlPOs), such as AlPO5, are analogues of siliceous (SiO 2 ) zeotypes; so benign zeotype analogues of the (Be,P,As)(O,OH) 2 phases described in this work but of the composition LiB(OH) 4 are readily conceived. For such a material the increased strength of hydrogen gas molecule adsorption on boron oxide surfaces compared with that on porous carbon is noteworthy [37] . Synthesis All of the samples were prepared from commercially available materials of reagent grade that did not require further purification. Warning: Be(OH) 2 is very toxic and may cause cancer by inhalation, H 3 AsO 4 is very toxic and is regarded as a carcinogen by all routes of exposure and may be fatal if ingested; for both these materials ensure adequate control measures are in place and the authors recommend that Be(OH) 2 is handled in a glove box. BET-As was synthesized via hydrothermal methods. Be(OH) 2 (0.374 g, 8.7 mmol), H 3 AsO 4 (0.33 ml, 4.34 mmol) and distilled H 2 O (3 ml) were added to a 23-ml Teflon vessel and stirred at room temperature for 30 min. Ethylamine (70 %, 2.83 ml, 0.0356 mol) was added to the mixture and the resulting gel allowed to age while gently stirring for a further 60 min. BET-P was synthesized using an equivalent composition replacing H 3 AsO 4 by the equivalent number of mmols of H 3 PO 4 . The mixture was then transferred to a Parr autoclave and heated at 160 °C for 168 h. The autoclave was allowed to cool naturally to room temperature and the white solid product was removed from the solution by vacuum filtration, washed with distilled water (20 ml) and ethanol (20 ml), and transferred to a drying oven at 80 °C for 12 h. The products BET-As and BET-P grew as sprays of thin crystal plates ( Supplementary Figs S7 and S8 ) BEE/BOT: (mixed phase product ~25% BEE and 75%BOT), Be(OH) 2 (0.055 g, 1.28 mmol) and H 3 AsO 4 (0.165 ml, 2.17 mmol) were added to a 23 ml Teflon vessel and stirred at room temperature for 30 min. Ethylamine (70%, 5 ml, 0.063 mol) was added to the mixture and the resulting gel allowed to age while gently stirring for a further 60 min. The mixture was then transferred to a Parr autoclave and heated at 160 °C for 192 h. The autoclave was allowed to cool naturally to room temperature and the white solid product was removed from the solution by vacuum filtration, washed with distilled water (20 ml) and ethanol (20 ml), and transferred to a drying oven at 80 °C for 12 h. The product was an intergrowth of needles of BEE and and larger tabular blocks of BOT ( Supplementary Fig. S9 ). Single crystal X-ray diffraction structure determination Single-crystal X-ray diffraction data were collected at 120 K on a Bruker Nonius KappaCCD diffractrometer (BEE) and at 100 K on a Rigaku FR-E+ Ultra High Flux Diffractometer (BOT, BET-P and BET-As), using Mo-Kα ( λ =0.71073 Å) radiation. Crystals normally formed as small needles (BOT), platelets (BET-P and BET-As) or tablets (BEE) and were very weakly scattering due to the high proportion of light atoms and large pore volumes. Several attempts to collect diffraction data at a synchrotron X-ray source were unsuccessful as the crystals decomposed in the intense beam during data collection. Data sets were therefore collected on very high flux laboratory X-ray systems described above with long data collection times—typically 10–24 h. Although diffraction data at higher angles (resolution <1.2 Å) were often weak, partly due to structural disorder in both the framework ( Be/As distribution) and template/water molecules, leading to relatively poor statistics for higher angle data, structure solution from these data produced excellent models for the frameworks in all cases. The disordered extra-framework electron density was modelled using the SQUEEZE method [38] . The structures were solved using the WinGX package [39] by direct methods using SHELX-97 (ref. 40 ) and XPREP [41] . Structure solution of BET-As BET-As grew as some of the largest crystals found in this work (up to 200×200×20 μm; Supplementary Fig. S7 )) and produced the best data statistically. The structure was solved in the monoclinic, P2 1 /m space group with β =89.970(2) deg; attempts to solve the structure in the higher symmetry orthorhombic Pnma (used for BET-P) gave significantly worse fits to the experimental data associated with the distribution of Be and As in the structure. Direct methods yielded positions for the majority of T atoms and subsequent Fourier maps were used to locate the remainder of the framework atoms, including Be-sites. All T sites were initially refined as mixed Be/As, although in later stages of the refinement those which gave Be site occupancies close to unity were set as Be atoms only. The model with framework atoms alone converged rapidly although with relatively high R factors, R1 typically 15–20%. SQUEEZE was used to identify pores within the structure and allocated scattering electron density to these. Subsequent refinement of the framework included anisotropic atomic displacement parameters (ADPs). For some framework oxygen atoms, especially those connected to T sites with mixed As/Be occupancy, high anisotropy in the ADPs was observed with elongation of the ellipsoid in one direction perpendicular to the T-O-T direction. This implied local positional disorder associated with the specific local occupancy of the two adjacent T sites (and reflecting the slighly different ideal T-O distances Be-O ~1.63 Å, As-O ~ 1.68 Å) and the possibility that this anion site may be O 2− or OH − (with each being expected to have slightly different distances to the adjacent T sites). Futher models were developed where the oxygen atoms with the highest anisotropy were placed over split sites corresponding to the extremes of the ADP ellipsoid. Although these models produced small improvements in R-factors and reduced ADPs for the split oxygen atom sites, they introduced significantly higher numbers of parameters into the refinement and did not necessarily represent an improved model to the range of local oxygen atom positions within the disordered framework. The structure reported is therefore that developed with full-site occupancies and a remaining few large ADPs on oxygen sites, representing the positional disorder described previously. A crystallographic information file (CIF) is provided for BET-As ( Supplementary Data 1) . Structure solutions of BET-P, BEE and BOT Crystals of BET-P grew as thin plates of largest dimensions 150×30×5 μm ( Supplementary Fig. S8 ) providing a crystallographic challenge due to their weak diffraction. The unit cell was determined to be similar to that of BET-As, although diffraction data could be fully indexed as orthorhombic ( β =90.0°). Full structure solution followed the same method as for BET-As. A CIF is provided for BET-P ( Supplementary Data 2 ). Crystals of BEE grew as fairly large transparent tablets of largest dimensions 100×50×20 μm ( Supplementary Fig. S9 ), although the monoclinic unit cell with V >9,000 Å 3 produced weak scattering at high diffraction angles. Full structure solution followed the same method as for BET-As; a CIF is provided for BEE ( Supplementary Data 3 ). Crystals of BOT grew as thin needles of largest dimensions 200×10×10 μm ( Supplementary Fig. S9 ). Full-structure solution followed the same method as for BET-As; a CIF is provided for BOT ( Supplementary Data 4) . Thermogravimetric analysis TGA was performed using a Polymer Laboratories STA 1500 simultaneous thermal analysis system. A 7-mg sample was heated in an alumina crucible to 230 °C at 2 °C min −1 under a flow of nitrogen gas. Variable temperature PXD PXD patterns were obtained by grinding the sample to a fine powder in an agate pestle and mortar. Room temperature PXD data were collected on a Siemens D5000 operating with Cu K α1 radiation. Variable temperature PXD patterns were collected on a Bruker D8 diffractometer operating with Cu K α1 radiation. The sample (100 mg) was heated to 300 °C in 100 °C steps and diffraction data collected between 2 and 20° 2 θ for 6 h at each temperature Infrared spectroscopy Infrared spectra were recorded using a Bio-Rad FTS 135 Fourier transform infra-red spectrometer equipped with a Golden Gate or using a Perkin-Elmer Spectrum One. Pore volume and surface area calculations Pore volumes, surface areas, largest cavity and pore-limiting diameters were calculated, using ZEOMICS [29] , for each of the BET, BEE and BOT topologies. Values are compared with those from the zeolites LTA, MOR and MFI [28] . For the new zeotypes reported in this work, specific pore volumes and surface areas are given for a pure siliceous framework, the composition as made(AX 2 ) and for a pure Be(OH) 2 material of that topology. BET surface area and pore volume measurements BET measurements were carried out using Micrometrics Gemini 2360 Surface area analyser with N 2 adsorption/desorption at 77 K. How to cite this article: Littlefield, B.T.R. and Weller, M.T. Lightweight nanoporous metal hydroxide-rich zeotypes. Nat. Commun. 3:1114 doi: 10.1038/ncomms2129 (2012).